Reprogramming within hours following nuclear transfer into mouse but not human zygotes Fertilized mouse zygotes can reprogram somatic cells to a pluripotent state. Human zygotes might therefore be useful for producing patient-derived pluripotent stem cells. However, logistical, legal and social considerations have limited the availability of human eggs for research. Here we show that a significant number of normal fertilized eggs (zygotes) can be obtained for reprogramming studies. Using these zygotes, we found that when the zygotic genome was replaced with that of a somatic cell, development progressed normally throughout the cleavage stages, but then arrested before the morula stage. This arrest was associated with a failure to activate transcription in the transferred somatic genome. In contrast to human zygotes, mouse zygotes reprogrammed the somatic cell genome to a pluripotent state within hours after transfer. Our results suggest that there may be a previously unappreciated barrier to successful human nuclear transfer, and that future studies could focus on the requirements for genome activation. The generation of animals by nuclear transfer [1] , [2] and the derivation of human embryonic stem cells [3] suggested that these two approaches might be combined to generate patient-specific embryonic stem cell lines. Because they would carry the patient's genotype, such stem cells might be useful for the production of autologous transplants [4] , [5] and for disease modelling [6] . Studies in mice have demonstrated the potential value of these combined approaches for treating severe combined immune deficiency and Parkinson's disease [7] , [8] . Although it is now possible to produce pluripotent stem cell lines with patient genotypes using defined reprogramming factors [9] , [10] , the equivalency of these cells to embryonic stem cells has been questioned. Several groups have found differences in gene expression, DNA methylation and differentiation propensity between iPS cells and ES cells [11] , [12] , [13] , [14] , [15] . Further, it has been suggested that induced pluripotent stem cells are not reprogrammed to the same extent that is observed in embryonic stem cells following nuclear transfer [16] . Therefore, it remains important to pursue human nuclear transfer as an alternative approach for producing stem cell lines. However, despite several attempts at human nuclear transfer [17] , [18] , [19] , [20] , [21] , [22] , [23] , [24] , these efforts have uniformly failed to produce stem cell lines. Instead, most studies reported developmental arrest during the cleavage stages. Consistent with this, the only stem cell line purportedly derived by human nuclear transfer [25] has subsequently been shown to originate from parthenogenesis rather than reprogramming of a somatic nucleus [26] . We have recently generated mouse embryonic stem cells by nuclear transfer into mitotic zygotes [27] , demonstrating that these cell types might also be a useful supplement to oocytes for human studies. Here we report programs for the acquisition of human preimplantation embryos, resulting in the donation of a significant number of human zygotes. When we performed nuclear transfer, development proceeded through the cleavage stages but arrested around the time of compaction. Our investigation into the causes of this blockade revealed that this developmental arrest may be the result of a failure to undergo transcriptional activation of the transferred somatic chromosomes. Thus, there is a barrier to reprogramming following human nuclear transfer that must be overcome before patient-specific embryonic stem cell lines can be derived. Donation of human zygotes Because we have had difficulty in accessing sufficient numbers of unfertilized oocytes to proceed with nuclear transfer studies [24] , we considered the possibility that human zygotes could serve as a source of recipient cytoplasm for nuclear transfer. We therefore initiated a program for recruitment of couples willing to donate their frozen zygotes for research. These protocols were approved by the participating academic institutions' committees on the use of human subjects in research, stem cell research oversight committees and the Western Institutional Review Board, an Associate of the Accreditation of Human Research Protection Programs. Between January 2007 and May 2010, 4,061 in vitro fertilization (IVF) embryos were donated by couples undergoing assisted reproduction. Though the majority of these were cryopreserved at either the cleavage- or blastocyst-stages, 461 (11.3%) were frozen at the one-cell-stage and therefore useful for nuclear transfer ( Fig. 1a ). These human zygotes were in excess of clinical need, but otherwise normal. 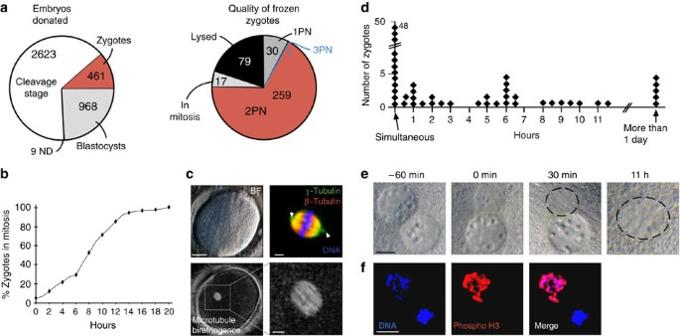Figure 1: Donation of human zygotes for stem cell research. (a) embryos donated for stem cell research. ND, not determined; PN, pronucleus. (b) Mitotic entry time of human zygotes (n=107) in hours after thaw. Nuclear envelope breakdown of at least one of the two pronuclei was defined as the time point of mitotic entry. Some zygotes were mitotic at the time of thaw. (c) mitotic spindle formation. Human zygote 30 min after nuclear envelope breakdown including brightfield image, microtubule immunohistochemistry (arrowheads point to the centrosome at both poles of the spindle) and spindle birefringence. Scale bar left panel 25 μm, right panels 5 μm. (d–f) asynchrony in nuclear envelope breakdown. (d) Hours between the breakdown of the first pronuclear envelope and the second. (e) Zygote with asynchronous pronuclear envelope breakdown. Numbers indicate the time from the breakdown of the first nuclear envelope. Scale bar, 10 μm. The location of mitotic chromatin is circled. (f) 1PN zygote stained for phosphorylation of Ser 27 on Histone H3, a marker of mitosis. Scale bar, 10 μm. Figure 1: Donation of human zygotes for stem cell research. ( a ) embryos donated for stem cell research. ND, not determined; PN, pronucleus. ( b ) Mitotic entry time of human zygotes ( n =107) in hours after thaw. Nuclear envelope breakdown of at least one of the two pronuclei was defined as the time point of mitotic entry. Some zygotes were mitotic at the time of thaw. ( c ) mitotic spindle formation. Human zygote 30 min after nuclear envelope breakdown including brightfield image, microtubule immunohistochemistry (arrowheads point to the centrosome at both poles of the spindle) and spindle birefringence. Scale bar left panel 25 μm, right panels 5 μm. ( d – f ) asynchrony in nuclear envelope breakdown. ( d ) Hours between the breakdown of the first pronuclear envelope and the second. ( e ) Zygote with asynchronous pronuclear envelope breakdown. Numbers indicate the time from the breakdown of the first nuclear envelope. Scale bar, 10 μm. The location of mitotic chromatin is circled. ( f ) 1PN zygote stained for phosphorylation of Ser 27 on Histone H3, a marker of mitosis. Scale bar, 10 μm. Full size image Nuclear transfer into mitotic human zygotes For successful reprogramming, we had previously cultured interphase mouse zygotes until they entered the first mitosis, and only then carried out nuclear transfer [27] . To investigate the reprogramming potential of human zygotes, we thawed 386 frozen human zygotes of which 307 (80%) were viable. Of these, 259 (84.4%) contained one maternal and one paternal pronucleus, as is typical for the first interphase in a normal, diploid zygote ( Fig. 1a ). These zygotes entered mitosis within 0–12 h after thawing ( Fig. 1b ), assembled a bipolar spindle ( Fig. 1c ), and, of 28 control zygotes, 9 (32%) developed to the blastocyst stage ( Supplementary Table S1 ). To better understand why not all zygotes developed to the blastocyst stage, and to exclude zygotes with low developmental potential from use in nuclear transfer experiments, we analysed the first mitosis in more detail. Another group has previously reported that progression through the first mitosis can accurately predict developmental potential [28] . Closer inspection of zygotes entering into mitosis revealed asynchrony of nuclear envelope breakdown. 34/82 zygotes (41%) did not simultaneously break down their two pronuclei, but instead did so with a delay of 30 min to up to 12 h ( Fig. 1d,e ). When 1PN (pronuclear) zygotes were stained for phosphorylation of Histone H3, a mitosis-specific modification of chromatin imposed by AuroraB kinase, we observed extensive phosphorylation on chromosomes of the pronucleus that had broken down, but not on chromatin of the pronucleus that had retained a nuclear envelope (three of three zygotes) ( Fig. 1f ). In addition, we observed a variety of other idiosyncrasies in human zygotes entering into mitosis. These included failure to condense the chromosomes ( Supplementary Fig. S1a ), a failure to completely dissolve nucleoli ( Supplementary Fig. S1b ) and a failure to assemble a mitotic spindle ( Supplementary Fig. S1c ). Zygotes exhibiting these abnormalities either arrested as single cells or eventually underwent fragmentation, and were excluded from use in nuclear transfer. The underlying cause of abnormalities we observed in frozen zygotes was not entirely clear. There was substantial variation in the age of frozen zygotes donated to us, with the oldest having been cryopreserved for as many as 20 years ( Supplementary Fig. S2 ). We do not favour the idea that these problems are a direct side effect of the freeze-thaw process, as 3/3 human zygotes frozen in mitosis were able to assemble a spindle within 30 min of thawing ( Supplementary Fig. S3 ), and because mouse zygotes frozen and thawed entered mitosis normally and could be used for nuclear transfer ( Supplementary Table S2 ). In the context of early nuclear transfer experiments, which controlled for micromanipulation of the human zygote, we found that the mitotic spindle could not properly direct cytokinesis if its position or orientation was disturbed ( Supplementary Figs S4-S6 ). We therefore devised a nuclear transfer strategy for human zygotes that was analogous to nuclear transfer into oocytes, thus overcoming this difficulty ( Fig. 2a ). 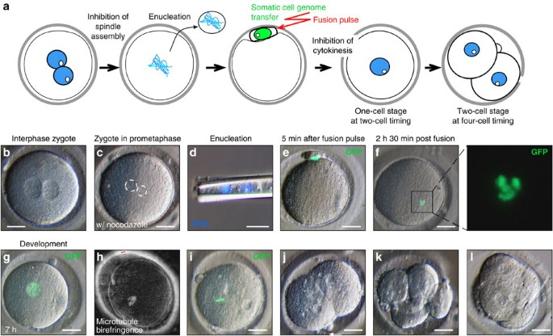Figure 2: Somatic cell nuclear transfer into human zygotes. (a) Schematic of nuclear transfer into human zygotes. (b) Zygote at 2PN stage in the presence of nocodazole. (c) Zygote at mitosis in the presence of nocodazole. Maternal and paternal haploid genomes are circled. (d) Paternal and maternal haploid genomes removed from the zygote. (e) Somatic cell nuclear transfer (green nucleus marked by H2B:GFP) by fusion, (f) chromosome condensation, (g) and 7 h after exit from mitosis. (h) Spindle assembly (i) chromosomes aligned at metaphase. (j) Cleavage, (k) six-cell stage, (l) morula-like, on d4 post fertilization. Scale bar, 25 μm. Figure 2: Somatic cell nuclear transfer into human zygotes. ( a ) Schematic of nuclear transfer into human zygotes. ( b ) Zygote at 2PN stage in the presence of nocodazole. ( c ) Zygote at mitosis in the presence of nocodazole. Maternal and paternal haploid genomes are circled. ( d ) Paternal and maternal haploid genomes removed from the zygote. ( e ) Somatic cell nuclear transfer (green nucleus marked by H2B:GFP) by fusion, ( f ) chromosome condensation, ( g ) and 7 h after exit from mitosis. ( h ) Spindle assembly ( i ) chromosomes aligned at metaphase. ( j ) Cleavage, ( k ) six-cell stage, ( l ) morula-like, on d4 post fertilization. Scale bar, 25 μm. Full size image In this novel nuclear transfer strategy, 69 human interphase zygotes were placed into a medium containing the microtubule-depolymerizing drug nocodazole ( Fig. 2b ). In all cases, these human zygotes proceeded into the first mitosis ( Fig. 2c ), but then, as intended, arrested due to inhibition of spindle assembly. This arrest in mitosis induced by nocodazole was stable but reversible and non-toxic ( Supplementary Fig. S7 ), allowing us to perform micromanipulation. Once mitotic entry occurred, we removed the zygotic chromosomes ( Fig. 2d ) and introduced interphase somatic donor nuclei ( Fig. 2e ). Skin cells of an adult healthy subject, or an adult type 1 diabetic subject served as nuclear donors. Because nuclear remodelling correlates with reprogramming in the rhesus monkey [29] , we monitored the transferred somatic chromatin hourly. We checked 46 of the 53 human zygotes (53/69, 77%) that survived these manipulations and found that 43 had undergone nuclear envelope breakdown and chromosome condensation within 6 h after transfer ( Fig. 2f ; Supplementary Fig. S8 ). Therefore, we concluded that early nuclear remodelling was generally successful. As intended, the unreplicated donor chromosomes could not satisfy the spindle checkpoint and, therefore, these zygotes remained in mitosis ( Supplementary Fig. S9 ). To induce mitotic exit, while inhibiting abnormal cytokinesis, we incubated zygotes in the cyclin-dependent protein kinase inhibitor purvalanol A, and the kinase inhibitor, 6-DMAP. Importantly, nocodazole, purvalanol A, and 6-DMAP are compatible with preimplantation development after nuclear transfer in mammalian species including the rhesus monkey [30] , [31] , [32] , [33] , suggesting that little, if any, toxicity would be expected when they are used. Within 4 h of drug treatment, 53/53 zygotes exited mitosis and entered the subsequent interphase ( Fig. 2g ). Zygotes were then monitored for entry into the subsequent mitosis, and within 30 h, 33/53 (62%) completed the second cell cycle. On mitotic entry, 33/33 assembled a spindle ( Fig. 2h,i ), proceeded through chromosome segregation, subsequent rounds of cleavage division ( Fig. 2j,k ), and 2/33 initiated compaction ( Fig. 2l ). However, we never observed further development to the blastocyst stage ( n =0/33). Genome activation fails after transfer into human zygotes Because we observed that all cleaving nuclear transfer cells generated using normal human zygotes (33/33) arrested at a similar developmental stage ( Fig. 3a ), we wondered whether there was a fundamental blockade to their development. Because of two observations, we considered the hypothesis that a failure to activate transcription was inhibiting development after nuclear transfer. Our first observation was that green fluorescence from the H2B–GFP protein transferred with the transgenic donor chromosomes was detectable at the first interphase. However, fluorescence intensity decreased with every cleavage and never returned (33/33 nuclear transfer specimen observed) ( Fig. 3b ). This observation suggested that even the H2B–GFP coding sequence under control of the strong CAAGS promoter was never again transcribed. In contrast, a similar transgene was routinely activated after mouse nuclear transfer [31] ( Fig. 3c ). Second, we found that development after nuclear transfer arrested at or shortly after the stage, when major transcriptional activation in the embryo normally occurs [34] , [35] . The steep increase in transcriptional activity in the normal embryo on day 3 after fertilization, or after the four-cell stage, was also termed zygotic genome activation (ZGA). 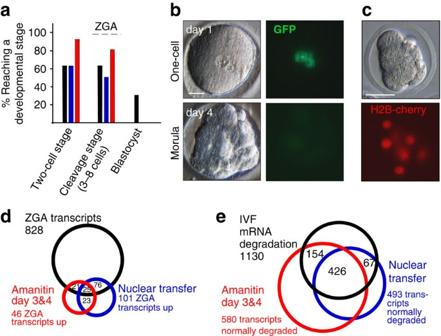Figure 3: Developmental potential and ZGA after nuclear transfer into human zygotes. (a) Developmental potential of control IVF human zygotes (black columns,n=28), zygotes after nuclear transfer (blue columns,n=53), and zygotes cultured in the presence of alpha-amanitin (red columns,n=23) displayed as the percentage of cells developing to and beyond the indicated developmental stage. (b) GFP expression after human nuclear transfer. (c) Transgene reactivation after mouse nuclear transfer. Shown are cells 2 days after nuclear transfer into mouse zygotes. (d) Genome activation after human SCNT. Venn diagrams of genes upregulated >fivefold in the indicated groups, (e) maternal mRNA degradation after human SCNT. Venn diagram of genes with transcript levels reduced by a factor of 5 or more in the indicated groups. NT, nuclear transfer. Scale bar, 25 μm. Figure 3: Developmental potential and ZGA after nuclear transfer into human zygotes. ( a ) Developmental potential of control IVF human zygotes (black columns, n =28), zygotes after nuclear transfer (blue columns, n =53), and zygotes cultured in the presence of alpha-amanitin (red columns, n =23) displayed as the percentage of cells developing to and beyond the indicated developmental stage. ( b ) GFP expression after human nuclear transfer. ( c ) Transgene reactivation after mouse nuclear transfer. Shown are cells 2 days after nuclear transfer into mouse zygotes. ( d ) Genome activation after human SCNT. Venn diagrams of genes upregulated >fivefold in the indicated groups, ( e ) maternal mRNA degradation after human SCNT. Venn diagram of genes with transcript levels reduced by a factor of 5 or more in the indicated groups. NT, nuclear transfer. Scale bar, 25 μm. Full size image We next asked whether there was a more global deficit in transcription following human nuclear transfer. To this end, we isolated RNAs from nuclear transfer and control embryos at equivalent developmental stages ( Supplementary Fig. S10a ) and then analysed their transcriptional profiles using microarrays. To understand the normal changes in transcription that occur during early stages of human cleavage development, we compared the profiles of unmanipulated one-cell zygotes collected on day 1 post IVF, to blastomeres of six to eight-cell embryos collected on day 3 (~72–84 h post IVF) and day 4 of development (~90–100 h post IVF). Relative to the maternal RNAs present in fertilized zygotes ( n =2 embryos), we found that 828 transcripts were significantly elevated (>fivefold, P <0.01, see Methods for statistical analysis) in all IVF samples ( n =19 embryos, 4 biological replicates). This result suggests there is substantial transcriptional activity already occurring at the six- to eight-cell stage, as has previously been reported [35] . In stark contrast, when the profiles of developmentally advanced nuclear transfer samples were examined ( n =2, 2 independent biological replicates, 6- to 8-cell stage), only 101 (12%) of these 828 transcripts were increased in their abundance relative to the 1-cell zygote ( Fig. 3d ) (>fivefold, P <0.01 for both samples). As a control to ensure that we could accurately monitor transcriptional changes in nuclear transfer blastomeres, we also monitored the decay of transcripts. At the cleavage stage, we observed that 1,130 maternal transcripts were subject to decay in all four control samples collected on day 3 and day 4 after IVF. The levels of each of these transcripts declined by a factor of 5 or more during normal development from the 1-cell stage to the 6- to 8-cell stage (<0.2-fold, P <0.01). Consistent with normal decay of a substantial fraction, but not all maternal RNAs, we found that 493 (44%) of these transcripts were also reduced at the cleavage stage following nuclear transfer (<0.2-fold, P <0.01) ( Fig. 3e ). To examine whether a somatic rather than an embryonic gene expression program was active after nuclear transfer, we defined a set of 2,153 transcripts that are transcribed at higher levels in the somatic donor cells than in human zygotes (>tenfold, P <0.001 for 2 somatic cell lines). Of the 2,153 transcripts, 85 (4%) were elevated in nuclear transfer samples (>fivefold higher levels than in zygotes, P <0.01 for 2 samples), wheras 350 (16%) were elevated in control IVF embryos (>fivefold higher levels than in zygotes, P <0.01 for 4 samples). Expression of these 350 transcripts after nuclear transfer would not require reprogramming, as they are already active in the somatic donor cell. Nevertheless, only 50 of them (14%) were elevated after nuclear transfer. This indicates that neither an embryonic nor a somatic transcriptional program was being expressed, and even genes that do not require reprogramming failed to be normally expressed after nuclear transfer. Inhibition of transcription induces cleavage stage arrest Our transcriptional analyses demonstrated that there was an unexpected failure to activate transcription at the appropriate time following human nuclear transfer. These results raise the possibility that development might arrest when the RNAs provided by the maternal stores are no longer sufficient to promote development. If this hypothesis is correct, then culture of normal fertilized zygotes in the transcriptional inhibitor alpha-amanitin should be sufficient to induce a developmental arrest identical to that observed following nuclear transfer. To test this idea, we cultured 23 zygotes for 5 days in the presence of the transcriptional inhibitor alpha-amanitin ( Fig. 3a ). We observed that 22/23 of these zygotes cleaved and 10/23 developed to the 6- to 8-cell stage ( Supplementary Table S1 ). However, no further development to the blastocyst stage occurred. In these arrested blastomeres, the number of transcripts with elevated levels was very similar to nuclear transfer samples: only 46 of the 828 transcripts (5.5%, P <0.01) normally rising in abundance over the first 3 days of development were increased >5-fold over the same time frame in alpha-amanitin-treated samples ( n =2 specimen, 2 biological replicates) ( Fig. 3d ). This result also suggests that as many of the 101 ZGA transcripts elevated in nuclear transfer blastomeres may be attributed to differential messenger RNA stability rather than active transcription. As observed after nuclear transfer, treatment with alpha-amanitin did not completely interfere with the degradation of maternal RNAs. We found that 590 of 1,130 (47%, <0.2-fold, P <0.01) transcripts that normally declined during cleavage also fell after alpha-amanitin treatment (samples collected on days 3 and 4 after IVF) ( Fig. 3e ). Therefore, pharmacological inhibition of transcription was sufficient to induce changes in mRNA levels and a developmental arrest identical to that observed after human nuclear transfer. Reprogramming within hours after transfer into mouse zygotes Although our experiments, thus far, suggest that there is a blockade to reprogramming using human zygotes that is not present when mouse zygotes are used, our human nuclear transfer protocol was technically distinct from the approach we had previously used for nuclear transfer using mouse zygotes [27] . To rule out the possibility that technical aspects of our human nuclear transfer procedure were preventing reprogramming, we used methods that we developed here for human nuclear transfer and asked whether they could support efficient development and reprogramming following nuclear transfer in mouse zygotes. To monitor the state of reprogramming, we used tail-tip fibroblasts carrying an Oct4::GFP transgene [36] . In striking contrast to our human experiments, we observed efficient development to the morula and the blastocyst stages (significance of difference mouse–human: χ 2 =0.002, Chi-square-test) ( Fig. 4a ; Supplementary Table S3 ). We also found that within less than 36 h, GFP became activated from the somatic chromosomes, suggesting that reprogramming of the Oct4 promoter had occurred and transcription initiated ( Fig. 4a ). This reprogramming following nuclear transfer was far more rapid than observed following induction of pluripotency in mouse fibroblasts using defined transcription factors [37] , [38] ( Fig. 4b ). We also controlled for the effects of cryopreservation by performing nuclear transfer into frozen-thawed mouse zygotes. These zygotes gave rise to blastocysts after nuclear transfer ( Supplementary Table S2 ). Thus, we can conclude that even when precisely the same nuclear transfer methods are used, mouse zygotes supported reprogramming, whereas human zygotes could not. 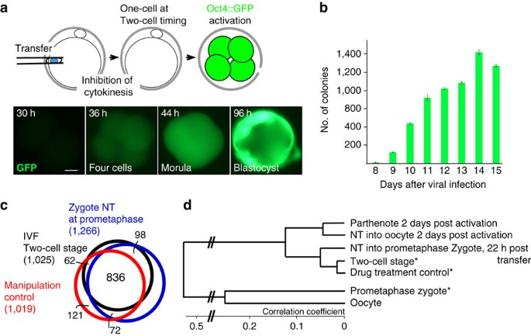Figure 4: Transcriptional reprogramming within hours after mouse nuclear transfer. (a) Oct4::GFP reprogramming after somatic cell nuclear transfer into mouse zygotes. (b) Number of Oct4–GFP+colonies during mouse iPS generation. Kinetics of Oct4::GFP reactivation in somatic cells after transduction with retroviruses carrying the reprogramming factors Oct4, Sox2, Klf4 and c-Myc. Day 8 is the eighthth day after the first exposure of somatic cells to viral vectors. (c,d) ZGA and reprogramming 22 h after nuclear transfer into mouse zygotes. (c) Venn diagram of transcripts elevated at the two-cell stage. (d) cluster diagram of the global gene expression profile after nuclear transfer into oocytes or zygotes. *From ref.31. Scale bar, 10 μm. Figure 4: Transcriptional reprogramming within hours after mouse nuclear transfer. ( a ) Oct4::GFP reprogramming after somatic cell nuclear transfer into mouse zygotes. ( b ) Number of Oct4–GFP + colonies during mouse iPS generation. Kinetics of Oct4::GFP reactivation in somatic cells after transduction with retroviruses carrying the reprogramming factors Oct4, Sox2, Klf4 and c-Myc. Day 8 is the eighthth day after the first exposure of somatic cells to viral vectors. ( c , d ) ZGA and reprogramming 22 h after nuclear transfer into mouse zygotes. ( c ) Venn diagram of transcripts elevated at the two-cell stage. ( d ) cluster diagram of the global gene expression profile after nuclear transfer into oocytes or zygotes. *From ref. 31 . Scale bar, 10 μm. Full size image To more broadly determine whether transcriptional initiation was occurring normally after mouse nuclear transfer into zygotes, we performed transcriptional profiling. In contrast to the situation in human development, where ZGA occurs at the four- to eight-cell stage [35] , in mouse, ZGA occurs at the two-cell stage [39] . Surprisingly, we found that transcriptional reprogramming was essentially complete by the end of the first cell cycle, or 22–24 h after nuclear transfer. Out of 1,025 transcripts that were upregulated between control mouse zygotes and the two-cell stage, 934 (91%) were also upregulated after nuclear transfer (>5×, P <0.01) ( Fig. 4c ). Chemically mock-treated control zygotes upregulated a similar number of transcripts (898/1,025, 88%). Remarkably, of 179 transcripts that were upregulated at the two-cell stage relative to the zygote (>fivefold, P <0.01) and that were not expressed in tail-tip fibroblasts, 151 were also upregulated after nuclear transfer, and 154 in mock-treated controls. This level of reprogramming was identical to that observed after nuclear transfer into mouse oocytes; the transcriptome of nuclear transfer embryos generated with zygotes clustered closely with unmanipulated two-cell embryos, and nuclear transfer embryos generated with oocytes clustered closely with parthenotes ( Fig. 4d ). To better understand the mechanism of reprogramming in mouse zygotes, we transferred somatic cells at various time points of mitosis. When somatic nuclei were transferred at prometaphase, chromosome condensation occurred within 2 h post transfer ( Fig. 5a,b ). In contrast, when nuclei were transferred at anaphase of mitosis, chromosome condensation did not occur and nuclear remodelling required 20 or more hours ( Fig. 5c–e ). Reprogramming and development after nuclear transfer into mouse zygotes was strictly dependent on nuclear remodelling by chromosome condensation. The transcriptome of zygotes transferred at anaphase clustered most closely with genome-less embryos, ( Fig. 5f ). Only 212/1,025 (20.7%) ZGA genes were normally expressed after nuclear transfer at anaphase ( Fig. 5g ), and of 179 ZGA genes silent in the somatic donor cell, only 23 (12.8%) were normally upregulated ( Supplementary Fig. S11a ). Furthermore, all embryos arrested at the two-cell stage when interphase nuclei were transferred, but development to the blastocyst stage was successful when mitotic genomes were transferred. ( Fig. 5h ; Supplementary Table S3 ). This observation raised the question whether a failure to condense somatic chromatin could be responsible for the transcriptional and developmental phenotype after nuclear transfer into human zygotes. However, this was not the case, as we found that 40/46 human zygotes underwent nuclear envelope breakdown and chromosome condensation within 3 h after transfer ( Supplementary Fig. S8 ). 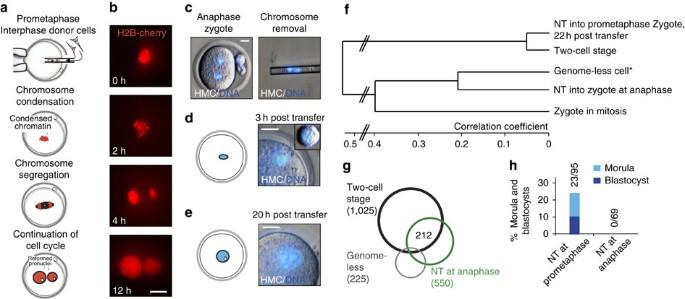Figure 5: Chromosome condensation is required for development and reprogramming after nuclear transfer into mouse zygotes. (a) Schematic for nuclear transfer into prometaphase and (b) corresponding images. Nuclei of fibroblasts at interphase are transferred into a zygote at prometaphase of mitosis. Chromosomes are marked with the red fluorescent fusion protein H2B-cherry. Shown is the mitotic progression after nuclear transfer. Time indicates the hours after nuclear transfer. Note the condensation of chromosomes and their separation into two groups, followed by formation of two pronuclei after inhibition of cytokinesis and entry into interphase. (c) Removal of the genome from a zygote at anaphase. (d) Nuclear morphology after transfer of interphase nuclei. Small inset: a somatic donor cell before transfer. Note that somatic donor chromatin is not condensed. (e) Nuclear remodelling is slow and requires about 1 day to restructure the nucleus into a large blastomere-like morphology. (f) Cluster analysis of gene expression after mouse SCNT. (g) Venn diagram of transcripts elevated 22–24 h after nuclear transfer at anaphase. (h) Nuclear transfer into zygotes at prometaphase or at anaphase of mitosis. Development to the morula and blastocyst stage as % of zygotes transferred with interphase somatic cell nuclei. Scale bar, 10 μm. *From ref.31. Figure 5: Chromosome condensation is required for development and reprogramming after nuclear transfer into mouse zygotes. ( a ) Schematic for nuclear transfer into prometaphase and ( b ) corresponding images. Nuclei of fibroblasts at interphase are transferred into a zygote at prometaphase of mitosis. Chromosomes are marked with the red fluorescent fusion protein H2B-cherry. Shown is the mitotic progression after nuclear transfer. Time indicates the hours after nuclear transfer. Note the condensation of chromosomes and their separation into two groups, followed by formation of two pronuclei after inhibition of cytokinesis and entry into interphase. ( c ) Removal of the genome from a zygote at anaphase. ( d ) Nuclear morphology after transfer of interphase nuclei. Small inset: a somatic donor cell before transfer. Note that somatic donor chromatin is not condensed. ( e ) Nuclear remodelling is slow and requires about 1 day to restructure the nucleus into a large blastomere-like morphology. ( f ) Cluster analysis of gene expression after mouse SCNT. ( g ) Venn diagram of transcripts elevated 22–24 h after nuclear transfer at anaphase. ( h ) Nuclear transfer into zygotes at prometaphase or at anaphase of mitosis. Development to the morula and blastocyst stage as % of zygotes transferred with interphase somatic cell nuclei. Scale bar, 10 μm. *From ref. 31 . Full size image Abnormal karyotypes do not cause transcriptional failure It has been suggested that mitotic abnormalities after primate nuclear transfer [40] cause karyotypic aberrations that contribute to developmental arrest. We therefore used fluorescence in-situ hybridization to investigate whether similar abnormalities occurred after human nuclear transfer and whether they might induce the transcriptional failures we observed. Although some chromosome abnormalities were observed, ( Supplementary Fig. S12 ), abnormalities were also found in IVF blastomeres ( Supplementary Table S4 ), many of which continue development to the morula and blastocyst stage. To directly test whether or not karyotypic abnormalities could be causing transcriptional failures, we intentionally induced aneuploidy in otherwise normal fertilized controls, and then monitored their transcriptional activity. To induce karyotypic abnormalities, we suppressed the first cleavage division, thus generating tetraploid cells with supernumerary centrosomes ( Fig. 6a ). These cells formed multipolar spindles at the next mitosis and directly cleaved into either three or four cells instead of two ( Fig. 6b ; Supplementary Table S5 ). As a consequence of the asymmetric segregation of chromosomes, the resulting blastomeres would be expected to have abnormal karyotypes. Despite their presumably abnormal karyotypes, we found that these blastomeres ( n =2, 1 replicate) initiated transcription (489/828 ZGA genes (59%) were upregulated at least fivefold, P <0.001) ( Supplementary Figure S13 ), and, therefore, their transcriptional profiles clustered closely together with normal IVF samples, and not with the nuclear transfer samples ( Fig. 6c ). Therefore, karyotypic abnormalities are not sufficient to explain the transcriptional failures we have observed following human nuclear transfer. Furthermore, as these zygotes were treated with nocodazole and the kinase inhibitors 6-DMAP and purvalanol A to inhibit cytokinesis, the same drugs as in our nuclear transfer protocols, they control for the effect of these drugs on transcriptional activation of the genome. We found that the transcriptional profile of these drug treated control zygotes clustered with untreated control embryos and clustered separately from nuclear transfer embryos ( Fig. 6c ). Therefore, the data suggests that the drugs used are not directly responsible for the transcriptional failures observed after somatic cell nuclear transfer. 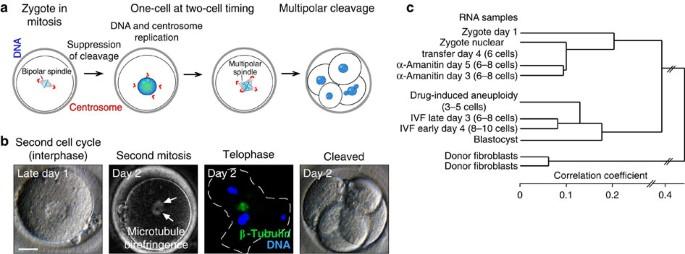Figure 6: Failure to initiate transcription is not caused by karyotypic abnormalities. (a) Induction of aneuploidy in human zygotes. Schematic showing development after suppression of cleavage at the first mitosis. (b) Development after suppression of cleavage at the first mitosis. Arrows point to a multipolar spindle as detected by microtubule birefringence. Immunohistochemistry at anaphase of mitosis shows the asymmetric segregation of chromatin to three poles (outer surface of the cleaving cell is outlined). Final panel: cleavage directly to 4 cells. NT=nuclear transfer. Days indicate the time post IVF. (c) Clustering of the transcriptome of the indicated samples. Scale bar, 25 μm. Figure 6: Failure to initiate transcription is not caused by karyotypic abnormalities. ( a ) Induction of aneuploidy in human zygotes. Schematic showing development after suppression of cleavage at the first mitosis. ( b ) Development after suppression of cleavage at the first mitosis. Arrows point to a multipolar spindle as detected by microtubule birefringence. Immunohistochemistry at anaphase of mitosis shows the asymmetric segregation of chromatin to three poles (outer surface of the cleaving cell is outlined). Final panel: cleavage directly to 4 cells. NT=nuclear transfer. Days indicate the time post IVF. ( c ) Clustering of the transcriptome of the indicated samples. Scale bar, 25 μm. Full size image Nuclear transfer into zygotes with supernumerary pronuclei Human zygotes fertilized by more than one sperm [41] , or which do not complete meiosis normally, are routinely discarded because of their abnormal chromosome content. We have shown that mouse polyspermic zygotes can serve as competent recipient cells [27] and, therefore, attempted to use 29 analogous human zygotes for nuclear transfer and developmental controls. As has been observed previously [42] , [43] , when the development of seven of these zygotes was monitored, they underwent abnormal cytokinesis ( Supplementary Table S5 ). We found that the unusual cleavage pattern that resulted was caused by the nucleation of tripolar or tetrapolar mitotic spindles with supernumerary centrosomes at the spindle poles ( Fig. 7a ). 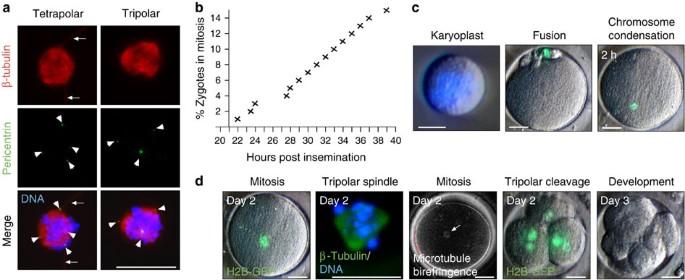Figure 7: Nuclear transfer into human polyspermic zygotes. (a) Immunocytochemistry of dispermic human zygotes at mitosis. Arrowheads point to pericentrin positive centrosomes, arrows to tubulin-positive sperm tails. Scale bar, 25 μm. (b) Entry of polyspermic zygotes into mitosis. Scale bars, left panel 5 μm, middle and right panels 25 μm. (c) Genome removed at mitosis, fusion with a somatic donor cell and chromosome condensation of the somatic cell genome 2 h post transfer are shown. (d) Cleavage and development after nuclear transfer into polyspermic zygotes. Time indicates the days post fertilization. The arrow points to a birefringent spindle. Scale bar, 25 μm. Figure 7: Nuclear transfer into human polyspermic zygotes. ( a ) Immunocytochemistry of dispermic human zygotes at mitosis. Arrowheads point to pericentrin positive centrosomes, arrows to tubulin-positive sperm tails. Scale bar, 25 μm. ( b ) Entry of polyspermic zygotes into mitosis. Scale bars, left panel 5 μm, middle and right panels 25 μm. ( c ) Genome removed at mitosis, fusion with a somatic donor cell and chromosome condensation of the somatic cell genome 2 h post transfer are shown. ( d ) Cleavage and development after nuclear transfer into polyspermic zygotes. Time indicates the days post fertilization. The arrow points to a birefringent spindle. Scale bar, 25 μm. Full size image We hoped that by arresting these zygotes in mitosis ( Fig. 7b ) and then removing their abnormal spindles, we might replace them with donor nuclei that would support normal cytokinesis. After we transferred nuclei into these mitotic zygotes, we again observed nuclear envelope breakdown and chromosome condensation ( Fig. 7c ). Following mitotic exit and inhibition of cytokinesis, entry into the second interphase occurred normally. However, in all instances, the next cleavage division was multipolar ( Supplementary Table S5 ), resulting in more than two, presumably aneuploid daughter cells and developmental arrest on day 3 after fertilization ( Fig. 7d ). Our results suggest that we were unable to remove supernumerary centrosomes during enucleation. Multipolar cleavage in human tetraploid zygotes was in striking contrast to both mouse and rabbit zygotes. In those species, tetraploid or polyspermic zygotes made a normal cleavage division, and efficiently developed to the blastocyst stage ( Supplementary Table S6 ). These results suggest that the centrosome has a more dominant role in directing spindle assembly and cytokinesis in human development than it does in other species. This observation has substantial ramifications for human nuclear transfer and suggests that, if more than one centrosome is present in the zygote after manipulations are completed, abnormal patterns of spindle assembly and cleavage will occur. Here we report our attempts to overcome the logistical and scientific obstacles impeding the production of patient-specific stem cell lines by nuclear transfer. While it has been difficult to recruit 'altruistic' oocyte donors [24] we did succeed in sourcing more than 400 normally fertilized eggs (zygotes) for our nuclear transfer studies. Development after nuclear transfer was normal through the cleavage stages, but, unlike IVF controls, all cleaving nuclear transfer cells arrested before or at the time of compaction with severe transcriptional abnormalities. An identical phenotype could be induced by inhibition of transcription in IVF controls, but not by the deliberate induction of karyotypic abnormalities, suggesting that transcriptional defects are more proximally responsible for the developmental arrest. Our findings are not the trivial result of a small sample size. Instead, our results of 160 nuclear transfer experiments and more than 175 control manipulations indicate that there is a robust species-specific blockade to reprogramming that must be overcome before human stem cell lines can be derived. Our work and those of others suggests that the developmental arrest we observed is not simply the result of using zygotes for nuclear transfer as a temporally similar arrest is commonly observed after nuclear transfer into to human unfertilized oocytes [18] , [20] , [25] . Although a single group has reported efficient transcriptional reprogramming after human nuclear transfer [20] , they compared somatic cells to nuclear transfer samples and their results are therefore confounded by the presence of maternal mRNAs, which were not appropriately accounted for by their analyses. Another group has generated a single blastocyst after transfer of embryonic stem cell nuclei into human oocytes [17] , but development arrested when fibroblasts were transferred using identical methods [18] . This suggests that development and activation of the transferred genome depend on the epigenetic state of the injected nucleus. In contrast to human zygotes, when we performed nuclear transfer into mouse zygotes, we found that reprogramming was essentially complete within hours and indeed within a single cell cycle. This result also points to a fundamental difference between reprogramming after nuclear transfer, and iPS reprogramming: at least in animals, nuclear transfer mediates an immediate transition from a somatic to a pluripotent gene expression pattern, whereas reprogramming by defined factors seems to be a gradual process, requiring days or weeks [37] , [38] . It is interesting to consider that this could explain why stem cells generated by nuclear transfer are indistinguishable [44] from stem cells derived from fertilized blastocysts, whereas in mouse [16] , [45] and human [12] , [15] , [46] , [47] , [48] iPS cell reprogramming may at times be less complete. Incomplete reprogramming and developmental defects after somatic cell nuclear transfer have been described in other vertebrate species [36] , [49] , [50] , [51] , [52] , [53] , [54] . For example, in bovine nuclear transfer embryos, 3.8% of genes were found to be incompletely reprogrammed [53] . This is comparable to the results reported here with mouse zygotes, where the majority of transcripts (>91%) are normally expressed within 24 h after nuclear transfer. In contrast, the transcriptional defects after nuclear transfer into human zygotes extend far beyond incomplete reprogramming of a few genes: the majority of transcripts, or more than 88%, were not normally expressed. Surprisingly, even genes that were active in the somatic donor cell were not normally expressed, suggesting a failure to properly activate the transferred somatic cell genome. The species-specific differences in transcription after nuclear transfer might be due to a property of the human egg, or of human somatic cells. Our results suggest that investigating the requirements for transcriptional activation of the donor cell genome may help to overcome the developmental arrest commonly observed after human nuclear transfer. Nuclear transfer into human zygotes Human zygotes were obtained using protocols reviewed and approved by the Committee on the Use of Human Subjects (IRB) and the Stem Cell Research Oversight Committee (ESCRO) at Harvard University. Human zygotes were thawed with Quinn's advantage thaw kit (Cooper Surgical). Zygotes were thawed in small groups, from 6–12 for a single experiment. On thawing, zygotes were washed and placed in microdrops of Global media under mineral oil, equilibrated overnight at 37 °C, 5% CO 2 . The 307 zygotes surviving the thaw were used as follows: 151 for nuclear transfer experiments, 77 for other experimental manipulations, 12 for immunohistochemistry and RNA analysis, 28 as developmental controls, and the remainder for developmental controls and the characterization of zygotic mitosis. The following nuclear transfer protocol emerged as the most practical: nocodazole was added 1–2 h post thaw at a concentration of 50 μg ml −1 . Lower nocodazole (Sigma) concentrations (0.1 μg ml −1 ) were ineffective for human zygotes ( Supplementary Fig. S14 , Supplementary Table S7 ), whereas vinblastine was effective even at low concentrations ( Supplementary Fig. S15 ). Without addition of nocodazole before spindle removal, most spindle material was removed with the zygotic genome ( Supplementary Fig. S16 ), resulting in developmental arrest and the formation of abnormal spindles at the next mitosis ( Supplementary Table S1 ). On entry into mitosis, zygotes were stained with Hoechst 33342 (2 μg ml −1 ) (Sigma) for 5–10 min in GMOPS-plus containing nocodazole. Zygotes were then placed on the heated stage in microdrops containing 10 μg ml −1 CytoB and 50 μg ml −1 nocodazole to generate a fluid cytoplasm. A hole was made in the zona pellucida with a XYClone Laser (Hamilton Thorne) using two to four 500–600 μs pulses. The DNA was removed using a fire-polished pipette to prevent lysis (73/116 zygotes, 63%, survived the enucleation step). Chromosomes were visualized by low-intensity UV illumination and/or Hoffman modulation contrast optics. Removal of genomic DNA was verified by the presence of Hoechst/DNA complex in the removed material and the absence in the zygote. A second hole was made and a somatic cell inserted below the zona pellucida. Somatic cells were allowed to reach confluency to induce cell cycle arrest (for both human or mouse somatic cells, this usually occurred within a week after passage), and maintained as confluent cultures until use for nuclear transfer (between 1 week to 2 months after reaching confluency). In some instances, cells were exposed to medium containing 0.5% serum for 1 day before use, for nuclear transfer. Fibroblasts obtained from a male adult T1D subject (ID#1,011) or an adult healthy male (ID#1,003) with a normal karyotype ( Supplementary Fig. S17 ) were used as nuclear donors. Fusion of the somatic cell was done using two DC pulses of 1.6 kV cm −1 of 20 μs width, using LF101 (Nepa Gene) in cell fusion medium containing 0.26 M mannitol, 0.1 mM MgSO 4 , 0.05% BSA, and 0.5 mM HEPES. 94 of 95 zygotes (99%) fused under these conditions, and none of them lysed. Using Piezo-mediated injection only 7/24, or 29% recovered from the lesion. On fusion, zygotes were returned to the incubator in Global culture medium. Chromosome condensation was monitored at least every hour using GFP fluorescence. After 2–3 h, chromosome condensation had occurred, and zygotes were stimulated to exit mitosis without cleavage using 2.5 mM 6-DMAP and 25 μM purvalanolA (Sigma P4484), in Global medium. After 4–5 h, when interphase nuclei were apparent, zygotes were thoroughly washed and then cultured in Global medium supplemented with 15% plasmanate. Incubation of zygotes in α-amanitin (Sigma) was done beginning 3–4 h after thaw at a concentration of 50 μg ml −1 . Our total survival rate for the total of 160 nuclear transfer manipulations was 108/160 or 67%. Microarray analysis For microarray analysis, total RNA was isolated using PicoPure RNA isolation kit (Molecular Devices), and RNA was amplified by two to three rounds of T7 transcription using the Illumina TotalPrep RNA Amplification Kit. Amplified RNA was hybridized to the Illumina Sentrix human gene expression BeadChip RefSeq 8 v3.0 and read by the Illumina Bead Array Reader. Analysis was done using the Illumina Genome Studio Program and Microsoft Excel. Data was normalized to average and a differential gene expression score calculated in comparison to one-cell zygotes as reference. Fold change to one-cell zygotes were calculated based on the average signal for a particular transcript using Microsoft Excel. The average fold change for two samples was calculated (for example, two samples on d3 post IVF, two samples on d4 post IVF, two samples treated with amanitin, two NT samples and so on). If the average fold change was >5 or <0.2, and the differential gene expression score was >22 or <−22, corresponding to a P -value of <0.01 for both samples, a transcript was considered differentially expressed. Differential gene expression score (Diffscore) is calculated by the Illumina Genome Studio program using an Illumina custom algorithm. A diffscore of >33 or <−33 corresponds to a P -value of <0.001. All P -values indicated in the manuscript were calculated in this manner. The 828 ZGA transcripts and the 1,130 maternal mRNA decay transcripts were at least 5× differentially expressed in the set of both d3 and d4 IVF data points, each consisting of two samples. Nuclear transfer into mouse zygotes and oocytes Nuclear transfer protocols developed on human zygotes were used for nuclear transfer into mouse zygotes. In brief, tail-tip fibroblasts used for nuclear transfer and iPS generation were obtained from adult B6jcBA-Tg (Pou5fI-EGFP)2Mnn/J mice. Mouse somatic cells were prepared for nuclear transfer as described above for human somatic cells. Zygotes and oocytes were obtained from BDF1 mice (Charles River). Zygotes were arrested in mitosis by nocodazole and had their genome removed shortly (5–10 min) after release from nocodazole with or without the use of Hoechst/low-intensity UV illumination. Nuclear transfer was done by two DC pulses of 1.6 kV cm −1 in fusion buffer (71/98 or 72% of tail tip cells fused and integrated into the recipient zygote). Cytokinesis was inhibited by incubation inhibited by the same combination of kinase inhibitors as used for nuclear transfer in human zygotes: 10 μM of the cyclin-dependent kinase inhibitor purvalanol A (Sigma P4484), 2 mM 6-DMAP (Sigma D2629), 0.5 μg ml −1 nocodazole, and optionally with the addition of 20 μM of the aurora B kinase inhibitor ZM 447439 (Tocris Bioscience) for 90–120 min. For nuclear transfer at anaphase, zygotes had their genome removed at anaphase (40–50 min post-nocodazole release) or, alternatively, the genome was removed at prometaphase, and zygotes were stimulated to enter anaphase as above (cytokinesis inhibitors purvalanol A, 6-DMAP and nocodazole) for 45–60 min before transfer. Control zygotes that had cytokinesis inhibited with these same cytokinesis kinase inhibitors efficiently developed to the morula and blastocyst stage (nine blastocysts and one morula of ten zygotes), suggesting that the combination of these drugs is not toxic to mouse preimplantation development. Nuclear transfer into mouse oocytes was done as follows: oocytes were obtained 14 h post hCG injection, their spindle–chromosome complex was removed in the presence of 5 μg ml −1 cytochalasinB. Tail-tip fibroblasts were transferred into enucleated oocytes by direct injection, and activated by 5 h incubation in 1 mM SrCl2 in ca-free MZCB and 5 μg ml −1 cytochalasinB to inhibit polar body extrusion, as described elsewhere [55] , [56] . Array data on nuclear transfer into genome-less zygotes were obtained from ref. 31 . Drug-treatment-only controls were arrested as zygotes with nocodazole, and cytokinesis was inhibited with the use of purvalanol A and 6-DMAP. For gene expression analysis, RNA was isolated from groups of ~20 cells, amplified by 2 rounds of T7 polymerase transcription and hybridized to Illumina arrays. Differentially expressed genes were defined as having a Diffscore of >22 or < than −22 in two samples of the same kind, and an at least fivefold difference in the average signal (average of both samples). Interphase zygotes were collected 25–28 h post hCG pulse, mitotic zygotes were obtained by nocodazole-mediated arrest until 33 h post hCG. iPS generation Plat-E packaging cells were transfected (Fugene, Roche) with retroviral plasmids for Oct4, Sox2, Klf4 or c-Myc and viral supernatant was collected, filtered, combined to contain virus of all four transcription factors, and placed on tail-tip cells obtained from adult B6jcBA-Tg (Pou5fI-EGFP)2Mnn/J mice for 3 consecutive days, as previously described (Ichida et al ., 2009). The first application of viral supernatant was counted as day 0. Immunostaining Zygotes, blastomeres and blastocysts were fixed in 4% paraformaldehyde overnight at 4 °C, permeabilized in PBS with 0.5%. Triton-X100 (PBS/T) for 20 min., blocked in blocking solution consisting of 0.1% PBS/T with 10% FBS overnight at 4 °C, incubated in primary antibody at 4 °C in blocking solution, then washed for 1 h at room temperature in 0.1% PBS/T, incubated with secondary conjugated antibody in 0.1% PBS/T at room temperature for 1 h, washed as above, stained with Hoechst 33342 for 5 min and used for confocal imaging. Oct4 antibody (Santa Cruz, sc5279) and Cdx-2 antibody (Biogenex) was used at a concentration of 1:200, and Brg-1 antibody (Santa Cruz sc-10768) was used at a concentration of 1:50. Conditions were maintained between different samples. BrdU labelling was done using the Amersham cell proliferation kit (RPN20). Cells were incubated into the labelling solution diluted 1:1,000 in KSOM for 18 h post transfer. Accession codes: Illumina array data have been deposited in the Gene Expression Omnibus database under accession number GSE28811 and GSE24631 . How to cite this article: Egli, D. et al . Reprogramming within hours following nuclear transfer into mouse but not human zygotes. Nat. Commun. 2:488 doi: 10.1038/ncomms1503 (2011).